Mesoporous monoliths of inverse bicontinuous cubic phases of block copolymer bilayers Solution self-assembly of block copolymers into inverse bicontinuous cubic mesophases is a promising new approach for creating porous polymer films and monoliths with highly organized bicontinuous mesoporous networks. Here we report the direct self-assembly of block copolymers with branched hydrophilic blocks into large monoliths consisting of the inverse bicontinuous cubic structures of the block copolymer bilayer. We suggest a facile and scalable method of solution self-assembly by diffusion of water to the block copolymer solution, which results in the unperturbed formation of mesoporous monoliths with large-pore (>25 nm diameter) networks weaved in crystalline lattices. The surface functional groups of the internal large-pore networks are freely accessible for large guest molecules such as protein complexes of which the molecular weight exceeded 100 kDa. The internal double-diamond ( Pn3m ) networks of large pores within the mesoporous monoliths could be replicated to self-supporting three-dimensional skeletal structures of crystalline titania and mesoporous silica. Porous polymer films and monoliths with internal bicontinuous nanoporous networks are increasingly important materials for applications such as desalination of water, ultrafiltration, chromatography, drug delivery, catalysis and nanotemplating [1] , [2] , [3] , [4] , [5] , [6] , [7] . In addition, polymer films and monoliths that have a three-dimensional (3D) crystalline array of internal nanoporous networks can serve as soft templates for creating mesoporous semiconductor crystals for highly efficient optical and optoelectronic materials and multifunctional hybrid materials [8] , [9] , [10] , [11] , [12] . In spite of recent advances in synthesizing porous polymers with internal bicontinuous porous networks [13] , [14] , [15] , [16] , [17] , [18] , [19] , [20] , microphase separation of block copolymers (BCPs) in bulk, followed by a selective removal of the labile polymer domains, remains a dominant method to create a cubic crystalline array of bicontinuous nanopores in polymer films and monoliths [21] , [22] . This method relies on the slow motion of BCPs in bulk, which might impede rapid synthesis of large monoliths with highly organized bicontinuous arrays of pores such as bicontinuous cubic structures [23] . Although solution self-assembly of BCPs has been widely used to create nanostructures with the desired morphology and functions [24] , [25] , this method generally yielded low-dimensional nanostructures, and, thus, has rarely been adopted as a method for the creation of highly ordered 3D periodic porous polymers. Peinemann, Abetz, and others [14] , [26] , [27] , [28] , [29] , [30] , [31] reported the synthesis of 3D porous polymers by non-solvent-induced phase separation of BCPs, which gives an integral asymmetric membrane with a highly ordered thin layer on top of a non-ordered sponge-like layer. Recently, Wiesner and co-workers [13] , [17] developed SIM 2 PLE (spinodal-decomposition-induced macro- and mesophases separation plus extraction by rinsing) method based on the phase separation of BCPs and spinodal decomposition between BCPs and oligomeric additives, rendering the resulting structures to be hierarchically porous polymer monoliths composed of ordered mesopores and randomly distributed macropores. Still, however, direct self-assembly of BCPs in solution into the dense inverse bicontinuous cubic (IBC) structures of the BCP bilayer in the form of films and monoliths has remained a challenge. Solution self-assembly of BCPs has shown the formation of inverse mesophases, which resulted in the formation of colloidal nano- and microparticles having internal bicontinuous pore networks [32] , [33] , [34] , [35] , [36] , [37] . The direct self-assembly of BCPs into IBC structures consisting of the BCP bilayers is an emerging method to create highly regular bicontinuous porous polymers without any aid of post processes to generate internal pore networks and surface functional groups [36] , [37] . We recently showed that the dendritic-linear BCPs composed of a dendritic block with peripheral hydrophilic poly(ethylene glycol) (PEG) chains and a glassy polystyrene (PS) hydrophobic block ( Fig. 1a ) preferentially self-assemble into inverse bicontinuous mesophases, in which the constituting BCP bilayers form the IBC structure, a 3D-flexed periodic structures of the membrane having zero mean curvature [32] , [36] . This self-assembly results in the formation of microscaled colloidal particles having internal non-interpenetrating networks of water channels weaved in a cubic crystalline order. The internal structures of the resulting colloidal particles (polymer cubosomes) consist of the IBC structure of the BCP bilayers, and show crystalline lattices over the long range including primitive cubic (P surface), double-diamond (D surface) and gyroid (G surface) symmetries. Peinemann and co-workers [37] also reported the formation of polymer cubosomes having internal P surface by self-assembly of poly(acrylic acid)- b -PS in dilute solution, which exhibited high sorption capabilities for proteins. This new synthetic strategy based on direct self-assembly of BCPs in solution could be greatly beneficial to the creation of porous polymers with 3D-ordered porous networks. However, the solution self-assembly of BCPs has rendered the resulting porous polymers to be colloidal particles rather than films and monoliths. 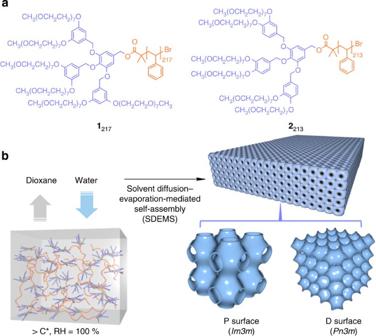Figure 1: SDEMS of dendritic-linear BCPs. (a) Chemical structures of dendritic-linear BCPs used in this study. The subscript indicates the average number of repeat units in the PS block. The weight fraction of the PEG domain is 9.3% for1217and 9.4% for2213. (b) Schematic illustration of SDEMS process and the monolith consisting of the IBC structures of the BCP bilayers. Figure 1: SDEMS of dendritic-linear BCPs. ( a ) Chemical structures of dendritic-linear BCPs used in this study. The subscript indicates the average number of repeat units in the PS block. The weight fraction of the PEG domain is 9.3% for 1 217 and 9.4% for 2 213 . ( b ) Schematic illustration of SDEMS process and the monolith consisting of the IBC structures of the BCP bilayers. Full size image We report here the direct solution self-assembly of amphiphilic dendritic-linear BCPs into mesoporous monoliths entirely composed of triply periodic IBC structures of the BCP bilayer. Utilizing the preferential self-assembly of dendritic-linear BCPs into inverse mesophases in solution [36] , we devise a simple and scalable method for the preparation of large mesoporous monoliths by self-assembly of the BCPs into the IBC structures, which is driven by the diffusion of a poor solvent (water) into the BCP solution under controlled humidity. This method allows the unperturbed growth of the porous monolith with an internal 3D cubic crystalline array of networks of large water channels (>25 nm) of a double-diamond lattice ( Pn3m ) with the desired surface functional groups. The internal network of the water channels may be used as a platform to accommodate guest molecules such as protein complexes, and the monolith is also demonstrated as a scaffold for the synthesis of 3D skeletal nanostructures of inorganic oxides with hierarchical porous networks. Solvent diffusion–evaporation-mediated self-assembly of BCPs In the routine practice for the self-assembly of dendritic-linear BCPs such as 1 217 and 2 213 ( Fig. 1a ) in dilute solution (cosolvent method), water, a poor solvent for the hydrophobic PS block, is gradually introduced to the BCP solution dissolved in dioxane, a common solvent for both of the polymer blocks. The addition of water destabilizes the PS blocks and consequently results in the aggregation of these PS blocks to form the core of the bilayer membrane, which has a corona composed of the PEG domain. This process inevitably requires physical agitation of the solution to ensure a homogeneous mixing of the two solvents, which renders the resulting self-assembled structures to be colloidal polymer cubosomes with microscaled sizes [36] . Therefore, the inverse bicontinuous structures formed in solution by self-assembly of BCPs remained colloidal particles rather than macroscopic objects such as films and monoliths. To avoid this formation of colloidal particles in solution, we devised a method to introduce water into the dioxane solution of the BCP without physical agitation or perturbation. We imagined that, under saturated humidity (relative humidity=100%), water vapour in the atmosphere would diffuse into the dioxane solution of 1 217 cast on a stationary substrate, with dioxane evaporating into the atmosphere. When the critical water content within the dioxane solution is reached (~15 vol%), the self-assembly of 1 217 would be initiated from the air–solution interface where the water content is presumably highest. We assumed that the formation of the IBC phases of the BCP would proceed downwards from the interface caused by diffusion of water. This method would ensure unperturbed growth of the monolith consisting of the IBC structure of the BCP because of the fast kinetics of self-assembly of 1 217 in solution. We tested our method, namely ‘solvent diffusion–evaporation-mediated self-assembly’ (SDEMS; Fig. 1b ), by placing a dioxane solution (12 wt%) of 1 217 cast on a glass substrate (0.5 mm wet film thickness) in a sealed humidity chamber (relative humidity=100%, 23 °C). After 1 h, the glass substrate was removed from the chamber and immersed into water to quench the assembly process by vitrification of the PS blocks. After removing dioxane by solvent exchange in water, we obtained the opaque monolithic film of 1 217 . Observed on scanning electron microscopy (SEM), this monolithic film revealed that the internal IBC structures consisting of the bilayer of 1 217 resided under the top layer (~10 μm thick) without any defined mesostructures ( Supplementary Fig. 1 ). When the same dioxane solution of 1 217 was placed in the same chamber filled with dry N 2 , we did not observe any formation of the IBC structures of the BCP. Instead, a transparent film without any mesoscaled internal structure was observed after solvent evaporation. We also observed the formation of polymer cubosomes instead of monoliths when the dilute dioxane solution of 1 217 (0.5–3 wt%) was used for the SDEMS ( Supplementary Fig. 2 ). This observation indicated that the formation of the inverse bicontinuous mesophase of 1 217 was the result of the self-assembly of the BCP in solution rather than the microphase separation of the BCP in bulk during the solvent evaporation. As the rate of dioxane evaporation under saturated humidity during the SDEMS process is directly related to the rate of the increase of water content, we expected that the kinetics of self-assembly of BCPs could be controlled by reducing the rate of dioxane evaporation. To prevent a premature quenching of the self-assembly of the BCP by a rapid increase of the water content, resulting in the formation of a featureless bulk of the BCP at the air–solution interface, we presaturated the humidity chamber with a mixture of water and dioxane (1:1 v/v) with an expectation that the dioxane vapour in the atmosphere would reduce the vapour pressure of the solvent, and thus slow down the rate of evaporation of the organic solvent. Under these conditions, a dioxane solution of 2 213 (12 wt%) was cast on a glass disk (2.5 cm diameter, 0.3 mm wet film height), and the coated disk was placed in a humidity chamber presaturated with a dioxane/water mixture (1:1 v/v) at 23 °C. After 1 h, the resulting disk was removed from the humidity chamber and immersed in excess water to remove residual dioxane, which yielded an opaque monolithic film on the substrate ( Fig. 2a inset). SEM images of the resulting monolith showed that the top layer of the monolith consisted of a perforated BCP bilayer, which exhibited an array of nanopores (~10 nm diameter) over the entire top surface (8.5 × 10 9 pores per cm 2 obtained by image analysis; Fig. 2a ). Below the top perforated bilayer, a highly crystalline inverse bicontinuous structure of polymer bilayers was observed over the entire thickness of the monolith (40 μm; Fig. 2b–e ). We also observed that the disordered domains and macroscopic defects gradually appeared within the monolith of 2 213 as the thickness of the monolith increased ( Fig. 2b ). We attributed this increased disorders within the monolith to the fact that the motion of polymer chains might be kinetically limited by the concentration gradient of water as the self-assembly progressed from the air–solution interface to the substrate by diffusion of water from the interface. 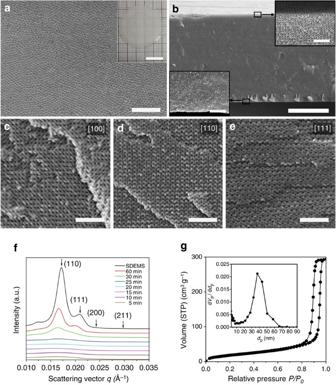Figure 2: Structural characterization of the monolith of 2213. (a) SEM images of the top layer of the monolith showing a perforated polymer layer having evenly distributed nanopores (~10 nm) in a long range. Scale bar, 1 μm. The inset shows a photograph of the polymer monolith of2213prepared on a glass substrate (2.5 cm diameter, scale bar, 1 cm.). (b) SEM image of the cross-section view of the monolith. Scale bar, 20 μm. The part highlighted by squares was magnified to show detailed morphology of the top and bottom edges (insets, scale bars, 500 nm.). (c–e) SEM images of the internal crystalline structures of the monolith of2213of a Pn3m lattice showing views at [100] (c), [110] (d) and [111] (e) directions. Scale bars, 300 nm (c–e). (f) SAXS results (5–60 min) by time-interval quenching of the self-assembled structures by immersion of the monoliths of2213in liquid N2. Black line indicates the SAXS pattern obtained by SDEMS without quenching by N2. The peaks were indexed toPn3msymmetry. (g) N2adsorption–desorption isotherms of the monolith of2213. The inset shows the BJH pore size distribution peaked at 37 nm. Figure 2: Structural characterization of the monolith of 2 213 . ( a ) SEM images of the top layer of the monolith showing a perforated polymer layer having evenly distributed nanopores (~10 nm) in a long range. Scale bar, 1 μm. The inset shows a photograph of the polymer monolith of 2 213 prepared on a glass substrate (2.5 cm diameter, scale bar, 1 cm.). ( b ) SEM image of the cross-section view of the monolith. Scale bar, 20 μm. The part highlighted by squares was magnified to show detailed morphology of the top and bottom edges (insets, scale bars, 500 nm.). ( c – e ) SEM images of the internal crystalline structures of the monolith of 2 213 of a Pn3m lattice showing views at [100] ( c ), [110] ( d ) and [111] ( e ) directions. Scale bars, 300 nm ( c – e ). ( f ) SAXS results (5–60 min) by time-interval quenching of the self-assembled structures by immersion of the monoliths of 2 213 in liquid N 2 . Black line indicates the SAXS pattern obtained by SDEMS without quenching by N 2 . The peaks were indexed to Pn3m symmetry. ( g ) N 2 adsorption–desorption isotherms of the monolith of 2 213 . The inset shows the BJH pore size distribution peaked at 37 nm. Full size image SEM images of the fractured monolith of 2 213 revealed the IBC crystalline structures of the BCP bilayers. These structures were assigned to a double-diamond lattice (D surface, Pn3m symmetry, lattice constant ( a )=51.7 nm) by synchrotron small angle X-ray scattering (SAXS) ( Fig. 2f ). Under the identical condition, 1 217 , an isomeric analogue to 2 213 that differs only in the structure of the benzyl ether dendritic block ( Fig. 1a ), self-assembled to form a monolith exhibiting similar morphology to the monolith of 2 213 ( Supplementary Fig. 3 ). The internal structure of the monolithic film of 1 217 was assigned to a primitive cubic lattice (P surface, Im3m symmetry, a =82.4 nm) coexisting with a double-diamond lattice (D surface, Pn3m symmetry, a =64.1 nm) by SAXS and SEM ( Supplementary Fig. 4 ). We, therefore, used the monolith of 2 213 for further structural characterization and our studies owing to the homogeneity of the internal crystalline lattice. The D surface structure also has been proposed to provide materials with interesting functions such as full bandgap photonic crystals and multifunctional hybrid materials such as a highly electrically conductive but poorly thermally conductive materials [11] , [12] . The formation of the internal IBC structure of the bilayer of 2 213 was traced using time-interval quenching of the self-assembled structure by immersion of the monolith in liquid N 2 , followed by a rapid exchange of the solvent by immersing the frozen structure in water. The rapid cooling of the self-assembled structure of 2 213 with liquid N 2 ensured that the BCP chains were in the glassy state, resulting in a minimal rearrangement of BCP chains while removing dioxane from the monolith. The quenched samples at each time interval were examined by SAXS and SEM. The results showed a gradual growth of the D surface of the BCP bilayer within the monolith over 1 h. ( Fig. 2f and Supplementary Fig. 5 ). From the SAXS results of the monolith of 2 213 prepared by SDEMS, we observed a weak peak appearing at low q region, which might result from the presence of disordered single continuous phases ( Fig. 2f ) [38] . Residual solvent molecules localized in the PS-rich domain would plasticize the PS blocks constituting the bilayer, and, therefore, could develop a pressure for the local grains of Pn3m symmetry to be rearranged to a single-diamond phase with some disorder [39] . As expected from the materials composed of glassy PS polymer blocks, the monoliths of dendritic-linear BCPs maintained the structural integrity at room temperature upon drying the solvents. The N 2 adsorption–desorption isotherms at 77 K revealed that the monolith of 2 213 exhibited a large surface area (73 m 2 g −1 ) and pore volume (0.45 cm 3 g −1 ) determined by Brunauer–Emmett–Teller (BET) analysis. The Barrett, Joyner and Halenda (BJH) analysis revealed the pore size distribution at 32 nm, which coincided with the observed pore dimension by SEM studies ( Fig. 2g ). The size and the thickness of the monolith were scalable as the BCP solution could be cast on a substrate of any size, and the thickness of the resulting monolithic film was proportional to the wet thickness of the polymer solution cast on a substrate. Using the SDEMS method, we were able to prepare a monolith of dendritic-linear BCPs with a thickness of 400 μm on a 25 cm 2 glass slide ( Supplementary Fig. 6 ). Surface functionalization of the mesoporous monoliths The bicontinuous cubic networks of large pores embedded within the IBC structure of the BCP bilayers could allow these porous polymer monoliths to be used as platforms for applications such as protein separation, biochemical transformation and nanotemplating [36] , [37] . To demonstrate the accessibility and usability of the internal networks of the water channels within the polymer monoliths, we introduced surface amino groups throughout the BCP bilayer by the co-assembly of 2 213 and NH 2 –PEG 45 –PS 210 , a linear BCP with an α-amino group at the hydrophilic PEG block under the SDEMS condition ( 2 213 /NH 2 –PEG 45 –PS 210 93:7 w/w in dioxane) [36] . The resulting surface-functionalized porous monolith exhibited the identical structural characteristics to the monolith of 2 213 , and showed an internal D surface structure ( Pn3m ) by SAXS and SEM ( a =63.2 nm; Supplementary Fig. 7 ). The surface amino groups of the monolith were converted to biotins to anchor streptavidin homo-tetramer labelled with fluorescein (54 kDa, Sigma) using the strong non-covalent interaction between biotin and streptavidin. On confocal laser scanning microscopy (CLSM), the resulting monolith showed a strong green fluorescence over the entire area (~1 cm 2 ) and thickness (~40 μm), which indicated that the fluorescein-labelled streptavidin was successfully bound to the surface biotin within the water channel networks. This streptavidin-bound monolith was immersed in a solution of the biotin-mCherry fluorescent protein (35 kDa; ref. 40 ), which yielded the monolith clearly showing cherry-coloured fluorescence owing to the binding of biotin-mCherry to the remaining binding sites of the surface-bound streptavidin ( Fig. 3a ). The axial intensity profile of fluorescence revealed the coexistence of streptavidin and biotin-mCherry fluorescent protein along the optical axis, which indicated the sequential binding of both proteins on the internal surface of the mesoporous networks within the monolith. The gradual decrease of fluorescence intensity along the depth of the monolith was derived from photobleaching during the measurement ( Fig. 3c ). This result demonstrated that the easy access of large guest molecules such as proteins and their complexes could easily access the internal networks of the large water channels of the polymer monolith. 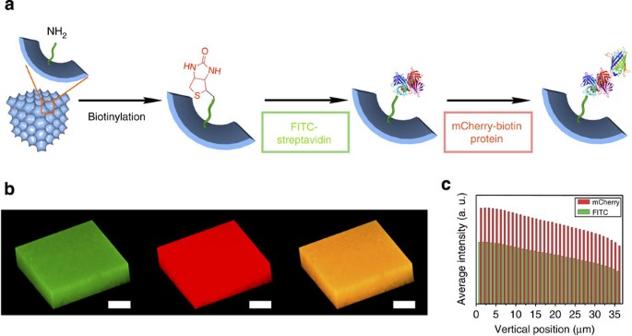Figure 3: Surface-functionalized internal large-pore networks of the mesoporous monolith. (a) Schematic illustration of surface functionalization of the monolith of2213/NH2–PEG45–PS210(93:7 w/w in dioxane) with protein complexes. The biotinylated monolith was complexed with fluorescein isothiocyanate-labelled streptavidin homo-tetramer. mCherry-biotin fluorescent protein was further assembled with the streptavidin on the surface of the monolith. Excess proteins was removed by rigorous washing procedures. (b) CLSM images of the biotinylated monolith of2213/NH2–PEG45–PS210(93/7 w/w) after binding of fluorescein isothiocyanate-streptavidin (λem=519 nm, left of panel). Subsequent binding of biotinylated-mCherry fluorescent protein (λem=610 nm, centre of panel) showed cherry-coloured fluorescence. Two images were merged (right of panel). The image was taken from 127 × 127 × 34 μm (width/height/depth) region near the top surface of the monolith. Scale bars, 40 μm. (c) Axial intensity profile of CLSM images along the optical axis was recorded from x, y, z image stacks, revealing the distributions of proteins. Figure 3: Surface-functionalized internal large-pore networks of the mesoporous monolith. ( a ) Schematic illustration of surface functionalization of the monolith of 2 213 /NH 2 –PEG 45 –PS 210 (93:7 w/w in dioxane) with protein complexes. The biotinylated monolith was complexed with fluorescein isothiocyanate-labelled streptavidin homo-tetramer. mCherry-biotin fluorescent protein was further assembled with the streptavidin on the surface of the monolith. Excess proteins was removed by rigorous washing procedures. ( b ) CLSM images of the biotinylated monolith of 2 213 /NH 2 –PEG 45 –PS 210 (93/7 w/w) after binding of fluorescein isothiocyanate-streptavidin ( λ em =519 nm, left of panel). Subsequent binding of biotinylated-mCherry fluorescent protein ( λ em =610 nm, centre of panel) showed cherry-coloured fluorescence. Two images were merged (right of panel). The image was taken from 127 × 127 × 34 μm (width/height/depth) region near the top surface of the monolith. Scale bars, 40 μm. ( c ) Axial intensity profile of CLSM images along the optical axis was recorded from x, y, z image stacks, revealing the distributions of proteins. Full size image Templated synthesis of skeletal inorganic structures These internal large-pore networks of the BCP monolith could be translated into the 3D self-supporting skeletal networks of functional organic and inorganic materials, which have structural symmetry inherited from the IBC structure comprising the BCP monolith ( Fig. 4 ). Therefore, we introduced liquid precursors of inorganic oxides such as titanium (IV) isopropoxide (Ti(OiPr) 4 ) into the D surface monolith of 2 213 (thickness 40 μm, 1 cm 2 area). Following the acid-catalysed crosslinking of Ti(OiPr) 4 to form TiO 2 , the resulting white monolith was sintered at 500 °C under ambient condition for 3 h to remove the BCP template ( Fig. 4 ; refs 41 , 42 ). The SEM and transmission electron microscopy (TEM) images of the resulting TiO 2 monolith ( Fig. 5a–c and Supplementary Fig. 8 ) showed that the monolith consisted of a skeletal replica of the water channel networks residing in the polymer monolith. SAXS analysis of the skeletal TiO 2 monolith revealed a diffraction pattern of the single-diamond phase ( Fd3m symmetry) ( Supplementary Fig. 9 and ref. 38 . Thermal treatment during calcination possibly affects structural constraints and causes a rearrangement of Pn3m to Fd3m owing to the increased mobility of polymer chains during calcination at the temperature well above glass transition temperature ( T g ) of PS block ( Figs 4 and 5 ; ref. 39 ). 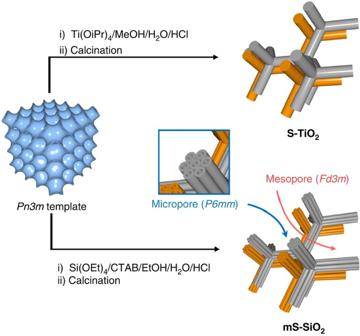Figure 4: 3D skeletal inorganic nanostructures replicated from the monolith of 2213. The monoliths of2213were used as templates for the fabrication of 3D skeletal porous inorganic nanostructures. The monoliths were immersed in each precursor solutions and excess solutions were removed before the calcination.mS-SiO2was schematically drawn to represent the hierarchically porous structure in which hexagonally ordered nanopores were incorporated into the skeletons consisting the self-supporting networks. Figure 4: 3D skeletal inorganic nanostructures replicated from the monolith of 2 213 . The monoliths of 2 213 were used as templates for the fabrication of 3D skeletal porous inorganic nanostructures. The monoliths were immersed in each precursor solutions and excess solutions were removed before the calcination. mS-SiO 2 was schematically drawn to represent the hierarchically porous structure in which hexagonally ordered nanopores were incorporated into the skeletons consisting the self-supporting networks. 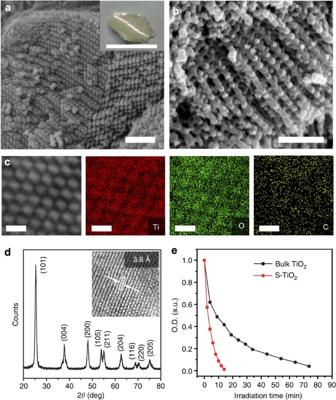Figure 5: Photocatalytic porous TiO2nanostructures replicated from the monolith of 2213. (a,b) SEM images ofS-TiO2synthesized within the mesoporous monolith of2213. Scale bars, 300 nm (a,b). The inset inashows a photograph ofS-TiO2monolith. (scale bar, 5 mm). (c) EDS mapping ofS-TiO2replicated from the monolith of2213. Scale bars, 50 nm. (d) X-ray diffraction data of the anatase TiO2skeletons consisting of the skeletal nanostructures. The inset shows a TEM image of the lattice structures of anatase TiO2skeletons. (e) Comparison of the photocatalytic activity ofS-TiO2with that of bulk TiO2under the same experimental conditions. Theyaxis indicates the optical density of the methylene blue solution, whereas thexaxis indicates the ultraviolet light irradiation time. Full size image Figure 5: Photocatalytic porous TiO 2 nanostructures replicated from the monolith of 2 213 . ( a , b ) SEM images of S-TiO 2 synthesized within the mesoporous monolith of 2 213 . Scale bars, 300 nm ( a , b ). The inset in a shows a photograph of S-TiO 2 monolith. (scale bar, 5 mm). ( c ) EDS mapping of S-TiO 2 replicated from the monolith of 2 213 . Scale bars, 50 nm. ( d ) X-ray diffraction data of the anatase TiO 2 skeletons consisting of the skeletal nanostructures. The inset shows a TEM image of the lattice structures of anatase TiO 2 skeletons. ( e ) Comparison of the photocatalytic activity of S-TiO 2 with that of bulk TiO 2 under the same experimental conditions. The y axis indicates the optical density of the methylene blue solution, whereas the x axis indicates the ultraviolet light irradiation time. Full size image The energy-dispersive X-ray spectroscopy mapping on TEM confirmed that the resulting 3D skeletal structures consisted of TiO 2 ( S-TiO 2 ) ( Fig. 5c ). The mean diameter of the constituting TiO 2 skeletons was determined to 15.5 nm by porosimetry, which was in line with the SEM and TEM images. We further revealed the characteristics of S-TiO 2 at the atomic scale by X-ray diffraction, which showed a pattern of the crystalline phase of TiO 2 in an anatase form. High-resolution TEM images of the skeletons of S-TiO 2 clearly showed a well-defined lattice space (0.38 nm) of the typical (100) crystalline plane of anatase TiO 2 ( Fig. 5d ). We investigated the photocatalytic activity of S-TiO 2 by monitoring the change in optical absorbance of methylene blue, which can be found as a water contaminant from dyeing processes [43] . Upon irradiation of a 3-ml methylene blue solution in the presence of S-TiO 2 (3 mg), the photodegradation of methylene blue was complete after 14 min, while the commercial TiO 2 nanoparticles (Sigma, <25 nm particle size) under the same experimental condition took nearly 80 min ( Fig. 5e ). The kinetics of the photodegradation reaction was plotted to a pseudo-first-order rate law using ln( C 0 / C )= kt , where k is the apparent rate constant and t is the irradiation time [44] . The average reaction rate constant of k for S-TiO 2 was 0.2764, min −1 , which was 6.4 times that of the reference anatase TiO 2 nanoparticles ( k =0.0434, min −1 ). BET analyses revealed that the surface area (80 m 2 g −1 ) of S-TiO 2 is greater than that of TiO 2 nanopowder (35 m 2 g −1 ; Supplementary Fig. 10 ). These results clearly indicated that the 3D skeletal nanostructure of S-TiO 2 provided an advantage to photodegradation of dyes arising from the large surface area and high accessibility to the catalytically active crystal planes. We could also realize the novel example of 3D hierarchically ordered structures with multiscale pores ( Figs 4 and 6a–c ). By infiltrating the monolith of 2 213 with tetraethylorthosilicate (Si(OEt) 4 ) in the presence of cetyltrimethylammonium bromide (CTAB), the skeletal mesoporous silica could be synthesized within the large channels of the porous polymer monolith [45] . After the crosslinking of Si(OEt) 4 and the calcination of the polymer template, we obtained the hierarchically mesoporous skeletal SiO 2 replica ( mS-SiO 2 ), of which the constituting silica skeletons (~18 nm in diameter) possessed the hexagonally ordered nanochannels ( a =3.58 nm, pore diameter~1.4 nm determined by SAXS) parallel to the long axis of the skeleton ( Fig. 6f,h ). SAXS results of the resulting mS-SiO 2 showed that the symmetry breaking from Pn3m to Fd3m occurred upon heating during calcination. SEM and TEM analyses revealed the random shifting of two non-intersecting skeletal networks by showing various projections of Fd3m in a similar manner to the report by Ho and co-workers [39] ( Fig. 6b–f and Supplementary Fig. 11 ). 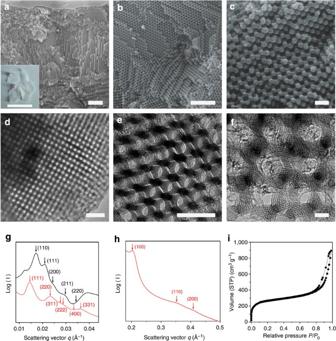Figure 6: Hierarchically porous SiO2skeletal nanostructures replicated from the monolith of 2213. (a) SEM image of the cross-section view ofmS-SiO2. The inset shows a photograph of the SiO2replica (scale bar, 5 mm). (b,c) SEM images ofmS-SiO2. Scale bars, 500 nm (a,b) and 100 nm (c). (d–f) TEM images ofmS-SiO2replicated from the monolith of2213. Scale bars, 100 nm (d,e) and 20 nm (f). (g) SAXS results of the monolith of2213(black,a=51.7 nm) used as the template andmS-SiO2(red,a=75.8 nm). The peaks were assigned toPn3m(black line) andFd3m(red line) symmetries, respectively. (h) SAXS result of hexagonally ordered nanopores residing in themS-SiO2(a=3.58 nm). (i) N2adsorption–desorption isotherms ofmS-SiO2. Figure 6: Hierarchically porous SiO 2 skeletal nanostructures replicated from the monolith of 2 213 . ( a ) SEM image of the cross-section view of mS-SiO 2 . The inset shows a photograph of the SiO 2 replica (scale bar, 5 mm). ( b , c ) SEM images of mS-SiO 2 . Scale bars, 500 nm ( a , b ) and 100 nm ( c ). ( d – f ) TEM images of mS-SiO 2 replicated from the monolith of 2 213 . Scale bars, 100 nm ( d , e ) and 20 nm ( f ). ( g ) SAXS results of the monolith of 2 213 (black, a =51.7 nm) used as the template and mS-SiO 2 (red, a =75.8 nm). The peaks were assigned to Pn3m (black line) and Fd3m (red line) symmetries, respectively. ( h ) SAXS result of hexagonally ordered nanopores residing in the mS-SiO 2 ( a =3.58 nm). ( i ) N 2 adsorption–desorption isotherms of mS-SiO 2 . Full size image The hierarchically porous structure of mS-SiO 2 was also confirmed by N 2 adsorption–desorption isotherms ( Fig. 6i ). The BET analysis of the isotherms showed an increased pore volume (1.38 cm 3 g −1 ) and surface area (953.7 m 2 g −1 ), which was threefold and 13-fold greater than the values of the mesoporous monolith scaffold, respectively. BJH analysis of N 2 adsorption–desorption isotherms of mS-SiO2 showed a broad pore distribution in a range of 6–20 nm, exhibiting the mean pore diameter of 5.9 nm ( Supplementary Fig. 12 ). The average diameter of hexagonally ordered smaller mesopores residing in the silica skeletons was estimated to be ~1.5 nm by the Horvath–Kawazoe model analysis ( Supplementary Fig. 12 ). This unique hierarchically porous structure could be beneficial for applications where large surface area and high accessibility to the structure are required simultaneously [46] . Solution self-assembly of amphiphilic BCPs into IBC mesophases is an emerging strategy to synthesize highly ordered mesoporous polymers with reticulated mesoscale porous networks without postsynthetic processes for pore generation. This direct self-assembly of BCPs in solution generated highly ordered triply periodic porous structures with the desired surface functional groups, which rendered these porous polymers potentially useful for separation, catalysis and nanotemplating. Our method (SDEMS) to induce self-assembly of BCPs in solution without physical agitation is based on the diffusion of a poor solvent for the PS block (water) into a solution in a common solvent to both polymer blocks. The diffusion of water at the air–solution interface gradually deteriorates the solvent quality towards the PS block, which propels the dendritic-linear BCPs to form bilayers in solution. In appearance, our method shares some resemblance to evaporation-induced self-assembly for the synthesis of mesoporous silica films [47] . Evaporation-induced self-assembly increases the surfactant concentration above the critical micelle concentration by gradually evaporating a common solvent, which allows the resulting mesoporous structures to be a form of films and monoliths. In our case, the diffusion of a poor solvent into the BCP solution is a key step to induce self-assembly because of the low critical micelle concentration values of BCPs. The rate of evaporation of a common solvent has to be suppressed to prevent a premature kinetic quenching of self-assembly of BCPs. Non-solvent-induced phase separation method by Peinemann, Abetz, and others [14] , [26] , [27] , [28] , [29] , [30] , [31] involves a quick phase separation of BCPs at the air–solution interface caused by evaporation of solvents, which was followed by a rapid solvent exchange with non-solvent within a phase-separated domain. SIM 2 PLE method by Wiesner and co-workers [13] , [17] is based on the phase separation of BCPs under solvent swollen conditions also rendered the resulting structures to be hierarchically porous polymer monoliths. Our method ensures that the self-assembly retain the characteristics of solution self-assembly, but only without physical agitation. The results and the demonstrations shown here substantiate that the highly ordered internal large-pore networks residing within the polymer monolith consisting of the IBC of the BCP bilayer could be valuable platforms for advanced separations and nanotemplating. We also point out that the results reported here suggest a new way to create highly ordered IBCs of BCP bilayers in a large scale by exploiting from the simple and fast solution self-assembly of BCPs in solution into inverse mesophases. General methods and materials Nuclear magnetic resonance spectra were recorded on a Varian VNMRS 600 spectrometer with CDCl 3 as a solvent. Molecular weights of BCPs were measured on an Agilent 1260 Infinity GPC system equipped with a PL gel 5 μm mixed D column (Polymer Laboratories) and differential refractive index detectors. Tetrahydrofuran (THF) was used as an eluent with a flow rate of 1 ml min −1 . A PS standard (Polymer Laboratories) was used for calibration. TEM was performed on a JEOL JEM-2100 and JEM-2100F microscope at an acceleration voltage of 200 kV. Sample specimens were prepared by placing a drop of the solution on a carbon-coated Cu grid (200 mesh, Electron Microscopy Sciences). After 30 min, remaining solution on a grid was removed with a filter paper, and the grid was air-dried for 18 h. SEM images were obtained on a FEI Nova NanoSEM 230 microscope and Hitachi S-4800 FE SEM at an acceleration voltage of 10 kV. The sample was placed on a conductive carbon layer and coated with Pt with a thickness of 3 nm by using a K575X Sputter Coater. CLSM was performed on a FluoView 1000 Confocal Microscope (Olympus). The Porous structures of the samples were analysed by a nitrogen adsorption experiment at 77 K using a BEL BELSORP-Max system. The surface areas and pore size distributions of the samples were calculated by using the BET equation and the BJH method, respectively. Small-angle X-ray scattering data were obtained on the SAXS beam line (PLS-II 9A) at Pohang acceleration laboratory (Pohang, Korea). Powder X-ray diffraction pattern was obtained on a D/MAZX 2500V/PC of Rigaku (Japan), the sample was ground before the measurement. Synthesis of BCPs All BCPs were synthesized and characterized by the literature procedures reported earlier ( Supplementary Figs 13 and 14 ; refs 36 , 48 ). The characterization of resulting BCPs are summarized in Supplementary Table 1 in Supplementary Information . SDEMS of BCPs In a typical procedure, 2 213 (20 mg) was dissolved in 1,4-dioxane (180 mg) in a 15-ml vial, and the resulting solution was kept at room temperature for 1 h before the use. A sealed humidity chamber was prepared by mixing 35 ml of 1,4-dioxane and 35 ml of water in a 100-ml vial, and then a cylindrical column to put a glass substrate was carefully added. A desired amount of the solution of 2 213 was carefully cast on the glass slide, which was rapidly placed on the column in the humidity chamber. The humidity chamber was then sealed for 1 h. After completing SDEMS, the glass slide covered with the monolith of 2 213 was immersed into excess water to quench the assembly process by vitrification of the PS block. The opaque monolithic film was then obtained after removing 1,4-dioxane by solvent exchange in water. Surface functionalization of the mesoporous monolith of 2 213 /NH 2 –PEG 45 –PS 210 The solution of 2 123 /NH 2 –PEG 45 –PS 210 (93:7 w/w in 1,4-dioxane) was applied under SDEMS condition. The monolith was then reacted with excess amount of NHS–PEG 4 –biotin (1,020 eq., Thermo Scientific) for 48 h, followed by washing with methanol and PBS (pH 7.4) several times. The monolith was incubated with excess amount of streptavidin homo-tetramer having fluorescein dye (54 kDa, Sigma) in PBS (pH 7.4) for 26 h. The excess streptavidin was removed by washing with PBS (pH 7.4). The streptavidin-bound monolith was immersed in a PBS solution of the biotin-mCherry fluorescent protein (35 kDa), followed by washing with PBS (pH 7.4). Synthesis of S-TiO 2 and mS-SiO 2 The monolith of 2 213 (thickness 40 μm, 1 cm 2 area) was impregnated with titanium (IV) isopropoxide, and then the acid-catalysed crosslinking of Ti(OiPr) 4 was allowed to form TiO 2 under HCl vapour for 2 h. The resulting white monolith was sintered at 500 °C under air condition for 3 h. Polymeric silica sol was prepared by refluxing TEOS, ethanol, water and HCl (molar ratios: 1:3:1:5 × 10 −5 ) at 80 °C for 1 h. Subsequently, CTAB solution (molar ratios, CTAB:EtOH:HCl=0.1:17:0.00395) was added to the silica sol. The monolith of 2 213 (thickness 40 μm, 1 cm 2 area) was soaked with the fresh sol, and aged at 40 °C for 1 h. The impregnated monolith was calcined under air condition at 520 °C for 4 h. Typical procedure for photodegradation reaction TiO 2 powder (3.0 mg) was suspended in aqueous solution (3 ml) of methylene blue (0.01 g/l) in a quartz cuvette. Before ultraviolet irradiation, the suspension was stirred in dark for 30 min to ensure the adsorption–desorption equilibrium of methylene blue onto the TiO 2 surfaces. The suspension was then irradiated under ultraviolet light ( λ =254 nm, 30 W). A portion of the reaction mixture was picked up from the mixture, centrifuged and analysed by ultraviolet-visible absorption spectroscopy. The kinetics of the degradation reaction was evaluated using the equation ln( C 0 / C )= kt , where k is the rate constant and t is the irradiation time. How to cite this article: Park, C. et al . Mesoporous monoliths of inverse bicontinuous cubic phases of block copolymer bilayers. Nat. Commun . 6:6392 doi: 10.1038/ncomms7392 (2015).